Sox2 antagonizes the Hippo pathway to maintain stemness in cancer cells The repressive Hippo pathway has a profound tumour suppressive role in cancer by restraining the growth-promoting function of the transcriptional coactivator, YAP. We previously showed that the stem cell transcription factor Sox2 maintains cancer stem cells (CSCs) in osteosarcomas. We now report that in these tumours, Sox2 antagonizes the Hippo pathway by direct repression of two Hippo activators, Nf2 (Merlin) and WWC1 (Kibra), leading to exaggerated YAP function. Repression of Nf2, WWC1 and high YAP expression marks the CSC fraction of the tumor population, while the more differentiated fraction has high Nf2, high WWC1 and reduced YAP expression. YAP depletion sharply reduces CSCs and tumorigenicity of osteosarcomas. Thus, Sox2 interferes with the tumour-suppressive Hippo pathway to maintain CSCs in osteosarcomas. This Sox2-Hippo axis is conserved in other Sox2-dependent cancers such as glioblastomas. Disruption of YAP transcriptional activity could be a therapeutic strategy for Sox2-dependent tumours. There is increasing evidence that tumorigenesis, metastasis and recurrence are fuelled by a minority of cancer cells which possess stem-cell like properties and thus have been termed cancer stem cells (CSC) [1] , [2] , [3] . CSCs are the only portion of the tumor population capable of initiating tumor growth, while continuously generating non-tumorigenic progeny cells that comprise the bulk of the tumor population. CSCs are predicted to be responsible for resistance to chemotherapy of many tumours, and thus methods of eradicating such cells could lead to tumour ‘sterilization’ and cure [4] , [5] , [6] . While the panoply of transcription factors and molecular networks that maintain stemness has been extensively studied in embryonic stem cells, much less is known about the factors that maintain CSC. Sox2, a transcription factor that is a key factor in maintaining stemness in embryonic as well as in adult stem cells, has been implicated in maintaining the undifferentiated tumorigenic state in cancers [7] , [8] , [9] , [10] , [11] . We have shown that this stem cell transcription factor maintains CSCs in osteosarcomas [12] , the most common bone malignancy in childhood and adolescence [13] . Molecular genetic analysis of sporadic and hereditary osteosarcomas in humans demonstrated that inactivation of the tumor suppressors Rb and p53 plays a role in their development [14] , [15] . Osteosarcomas arise from mesenchymal stem cells (MSC) or early osteoprogenitors and are the second most frequent tumour in patients with hereditary retinoblastoma. Individuals with a germ line mutation in the RB-1 gene have a 500-fold increased risk of osteosarcoma [16] , [17] . Osteosarcomas originate at high frequency in mice following conditional knock-out (KO) of the Rb-1 and p53 genes in the osteoblastic lineage [14] , [15] . Sox2 is highly expressed in human and murine osteosarcomas (mOSs), and is greatly enriched in cells capable of forming spheres in suspension culture (called osteospheres or sarcospheres) thought to represent a population of self-renewing stem-like cells. Osteosarcoma cells have a disrupted osteogenic differentiation programme, and cells depleted of Sox2 lose their tumorigenic properties and regain the ability for osteogenic differentiation. mOSs contain at least two populations of cells, with high Sox2 and high stem cell antigen (Sca-1) expression marking cells with stem cell properties that are blocked in osteogenic differentiation, while low Sca-1, low Sox2-expressing cells as well as Sox2-depleted cells can differentiate into mature osteoblasts. These findings support the hypothesis that Sox2 marks a population of osteosarcoma stem cells that, despite other mutations, maintain a requirement for Sox2 for tumor initiation or maintenance [12] . Osteosarcomas are also frequent in mice with a heterozygous knockout of the Nf2 (neurofibromin 2, merlin) gene [18] . Nf2 is a FERM (F for 4.1 protein, E for ezrin, R for radixin and M for moesin) family protein that plays a critical role in the establishment of adherent junctions and is an important mediator of contact inhibition [19] . It is a component of the Hippo signalling cascade whereby it acts as a scaffold to mobilize the core Hippo kinases. The Hippo pathway regulates organ size by inhibiting cell proliferation and is conserved across species [20] , [21] . Deregulation of the Hippo pathway has been implicated in several cancers pointing to its tumour suppressive role in restraining the function of its downstream effectors, YAP and TAZ [22] , [23] , [24] , [25] . When the Hippo pathway is active, the two transcriptional co-activators, YAP and TAZ are phosphorylated and sequestered in the cytoplasm, thereby inhibiting their transcriptional activity [26] . When the pathway is inactive, the two co-activators can readily localize to the nucleus, bind to the TEAD group (TEAD 1-4) of DNA-binding proteins and activate gene transcription [27] . The upstream components of the Hippo pathway (Nf2, Mst1/2, Sav1, Lats1/2 and Mob1A) have tumour suppressive activity, while the downstream components (YAP, TAZ and TEAD) behave as oncogenes. In this report, we show that Sox2 disrupts the Hippo pathway in osteosarcomas to maintain an undifferentiated tumorigenic state characterized by high YAP expression. This is achieved by direct transcriptional repression of Nf2 (Merlin), and WWCI (Kibra), and increased YAP expression. Downregulation of YAP expression or upregulation of Nf2 decreases the ability of osteosarcoma cells to form osteospheres and promotes osteogenic differentiation. Notably, YAP overexpression as well as Nf2 or WWC1 downregulation can restore osteosphere formation in Sox2-depleted cells. Our findings identify a novel Sox2-Hippo axis that maintains osteosarcomas in a stem-like state. High YAP and low Nf2 and WWC1 expression are observed in a large number of human osteosarcomas, and we find that this regulatory circuit is conserved in other tumour types that show high Sox2 expression, such as glioblastoma multiforme (GBMs). Thus, we identify a direct link between Sox2 and the Hippo tumour-suppressive programme in CSCs. Our studies indicate that restoring Hippo signalling or interfering with YAP function could be a novel therapeutic strategy in cancers with Sox2-mediated Hippo pathway inactivation. Gene expression profiles of Sox2-knockdown mOS cells We compared the gene expression profiles of two mOS cell lines, mOS-482 and mOS-379, with that of their corresponding Sox2-depleted (by Sox2 shRNA) counterparts that are no longer tumorigenic and can easily differentiate into the osteoblastic lineage [12] . Both cell lines were derived from spontaneous osteosarcomas that arose in a mouse model in which Rb and p53 are deleted in the osteogenic lineage. Using microarray hybridization (Affymetrix 430 A2.0) and differential expression analysis (fold change>1.66, P <0.05 by t -test) ~23% (5,284/22,690) entities were significantly altered ( Fig. 1a ). Gene ontology analysis (functional annotation clustering) was performed on significantly up- and downregulated genes to yield insights into the biological functions regulated by Sox2 in this setting ( Fig. 1a ). The microarray data were also subjected to unbiased Gene Set Enrichment analysis against curated gene sets. 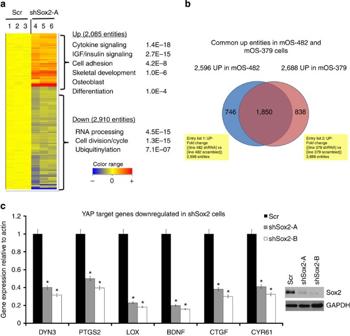Figure 1: Gene expression analysis of Sox2-regulated genes in osteosarcomas. (a) Heat map of hierarchically clustered genes in mOS-482 cells expressing scrambled (Scr) or Sox2 shRNA-A (shSox2-A). The expression level of all 22,670 entities is shown in triplicate samples. Significantly upregulated (red) and downregulated (blue) GO terms and enrichmentPvalues by DAVID are shown. (b) Venn diagram showing intersection of differentially upregulated genes in Sox2-depleted mOS-379 and mOS-482 cells. Nf2 and WWC1 were identified in the overlap. (c) qRT-PCR of mRNA expression of YAP-TEAD transcriptional target genes in Sox2-depleted mOS-482 cells using two independent Sox2 shRNAs (shSox2-A and shSox2-B). Gene expression was normalized relative to actin. *P<0.05 by ANOVA, Error bars, mean ± s.d. western blot of Sox2 expression is shown. Figure 1: Gene expression analysis of Sox2-regulated genes in osteosarcomas. ( a ) Heat map of hierarchically clustered genes in mOS-482 cells expressing scrambled (Scr) or Sox2 shRNA-A (shSox2-A). The expression level of all 22,670 entities is shown in triplicate samples. Significantly upregulated (red) and downregulated (blue) GO terms and enrichment P values by DAVID are shown. ( b ) Venn diagram showing intersection of differentially upregulated genes in Sox2-depleted mOS-379 and mOS-482 cells. Nf2 and WWC1 were identified in the overlap. ( c ) qRT-PCR of mRNA expression of YAP-TEAD transcriptional target genes in Sox2-depleted mOS-482 cells using two independent Sox2 shRNAs (shSox2-A and shSox2-B). Gene expression was normalized relative to actin. * P <0.05 by ANOVA, Error bars, mean ± s.d. western blot of Sox2 expression is shown. Full size image Both types of analyses revealed that cell cycle progression and mitosis-related genes were downregulated on Sox2 deletion, consistent with the lower rate of proliferation of Sox2-depleted cells. Downregulated gene sets include RNA processing and protein ubiquitination suggesting that Sox2 promotes these biological processes. In the genes upregulated by Sox2 deletion, there was a significant enrichment of genes related to osteogenic differentiation and skeletal ossification, consistent with the increased ability of these cells to undergo osteogenic differentiation. Upregulated gene sets also included chemokine secretion, IGF/insulin signalling, adhesion and G-protein signalling ( Fig. 1a and Supplementary Fig. 1 ), pathways important for osteoblastic differentiation [28] . We overlapped the gene expression changes from mOS-482 cells with mOS-379 cells (that are heterozygous for p53 deletion) [12] . While the mOS-379 cells showed less marked fold changes, the results from GO analysis of overlapped gene expression changes were consistent with those seen in mOS-482 cells( Fig. 1b ). The intersection of differentially regulated genes in both cell lines with those obtained in our Sox2 Chip-Seq experiments in osteoprogenitor cells [29] provided a stringent set of potential direct targets of Sox2. Because of our observed Sox2 regulation of YAP in MSC and osteoprogenitors [29] , and the fact that the Hippo pathway is tumour suppressive in a variety of cancers, we examined in detail the expression of genes that are components or targets of Hippo signalling. The expression of several YAP/TEAD target genes was repressed in Sox2-depleted cells ( Fig. 1c ). Furthermore, the 159 repressed genes identified as putative direct Sox2 target genes included two activators of the tumour-suppressive Hippo pathway, Nf2 (refs 19 , 30 ) and WWC1 (ref. 31 ). These results prompted us to study the regulation of these components of the Hippo pathway in osteosarcomas. YAP, Nf2 and WWC1 are deregulated in osteosarcomas In MSCs as well as in the more differentiated osteoprogenitors, Sox2 strongly induces the expression of YAP, by binding to the YAP gene and activating its transcription [29] . YAP induction contributes to the inhibition of the pro-differentiation Wnt pathway and to maintain ‘stemness’ in MSC and osteoprogenitors. YAP overexpression counteracts the ability of the Lats kinases to promote its phosphorylation, resulting in increased association of YAP with the TEAD transcriptional cofactors, thereby counteracting the repressive effects of the Hippo pathway [26] . We examined the expression of YAP, Nf2 and WWC1 protein in a large number of murine and human osteosarcoma cell lines that we had previously reported to express high levels of Sox2. YAP protein was uniformly increased, although to a varying extent, in all the cells tested, while Nf2 and WWC1 were reduced compared with normal osteoblasts ( Fig. 2a ). Accordingly, immunohistochemical analysis of sections of spontaneous osteosarcoma arising in the p53/ Rb double-knockout mouse model detected high Sox2 and YAP in the tumour cells, while areas of more differentiated cells were unstained ( Fig. 2b ). Importantly, a meta-analysis of YAP, Nf2 and WWC1 mRNA expression in a panel of human osteosarcomas also showed that YAP expression is higher in osteosarcomas, whereas the expression of the two activators of the Hippo pathway is downregulated in this tumour type [32] ( Fig. 2c ). The expression of TAZ, the YAP paralogue [33] , was also elevated in several osteosarcoma tumour samples, but not as consistently as that of YAP (meta-analysis not shown; see discussion), and TAZ is not expressed in the mOS-482 and mOS-379 osteosarcoma cells ( Supplementary Fig. 2a ). 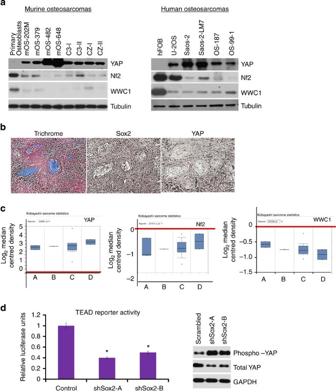Figure 2: Deregulation of the Hippo pathway in osteosarcomas. (a) Western analysis of YAP, Nf2 and WWC1 in murine and human osteosarcoma cell lines. (b) YAP and Sox2 expression in a spontaneous osteosarcoma in a bone-specific p53/Rb-knockout mouse. Massie’s trichrome stain (left panel) and immunohistochemistry with Sox2 (middle panel) and YAP (right panel) antibodies demonstrate that differentiated areas of the tumour (stained blue for collagen) have low expression of Sox2 and YAP. Scale bar, 100 μm. (c) mRNA expression of YAP, Nf2 and WWC1 in human osteosarcomas tumour samples. Box plot shows mRNA expression of YAP, Nf2 and WWC1, as compared with control (red line). A=chondroblastic osteosarcoma; B=fibroblastic osteosarcoma; C=osteoblastic osteosarcoma; and D=telangietactic osteosarcoma. Data used in this analysis were downloaded fromwww.oncomine.org. (d) Expression of the 8X-GTIIC(TEAD) luciferase reporter in mOS-482 cells expressing either scrambled or two independent Sox2 shRNAs -A and B. Cells were transfected with a TEAD-Luciferase (Firefly) reporter. Luciferase activity was normalized to Renilla luciferase. *P<0.05 by ANOVA. Error bars represent mean ± s.d. (e) Western analysis of phospho- and total YAP in mOS-482 cells expressing scrambled or two independent Sox2 shRNAs-A and B. The anti-phospho YAP antibody recognizes the phosphorylated S127 residue. Figure 2: Deregulation of the Hippo pathway in osteosarcomas. ( a ) Western analysis of YAP, Nf2 and WWC1 in murine and human osteosarcoma cell lines. ( b ) YAP and Sox2 expression in a spontaneous osteosarcoma in a bone-specific p53/Rb-knockout mouse. Massie’s trichrome stain (left panel) and immunohistochemistry with Sox2 (middle panel) and YAP (right panel) antibodies demonstrate that differentiated areas of the tumour (stained blue for collagen) have low expression of Sox2 and YAP. Scale bar, 100 μm. ( c ) mRNA expression of YAP, Nf2 and WWC1 in human osteosarcomas tumour samples. Box plot shows mRNA expression of YAP, Nf2 and WWC1, as compared with control (red line). A=chondroblastic osteosarcoma; B=fibroblastic osteosarcoma; C=osteoblastic osteosarcoma; and D=telangietactic osteosarcoma. Data used in this analysis were downloaded from www.oncomine.org . ( d ) Expression of the 8X-GTIIC(TEAD) luciferase reporter in mOS-482 cells expressing either scrambled or two independent Sox2 shRNAs -A and B. Cells were transfected with a TEAD-Luciferase (Firefly) reporter. Luciferase activity was normalized to Renilla luciferase. * P <0.05 by ANOVA. Error bars represent mean ± s.d. ( e ) Western analysis of phospho- and total YAP in mOS-482 cells expressing scrambled or two independent Sox2 shRNAs-A and B. The anti-phospho YAP antibody recognizes the phosphorylated S127 residue. Full size image Taken together these data suggest that a profound suppression of the Hippo pathway characterizes murine and human osteosarcomas, with downregulation of two essential activators (WWC1 and Nf2) and upregulation of YAP, a downstream effector that is restrained by Hippo signalling. Activation of the Hippo pathway leads to phosphorylation and nuclear exclusion of YAP resulting in repression of YAP/TEAD target genes. Consistent with the notion that the Hippo pathway is antagonized in mOS cells, and activated in Sox2-depleted cells, we found that the expression of several YAP/TEAD target genes ( DYN3 , PTGS2 , Lox , BDNF , CTGF and CYR61 ) is reduced in Sox2-depleted cells ( Fig. 1c ) [29] , [34] . To further test this hypothesis, we introduced into parental or Sox2-depleted mOS cells a YAP/TEAD-responsive reporter plasmid [35] and measured its activity in the two cell types. The activity of the reporter plasmid was high in the parental mOS cells and much lower in their Sox2-depleted non-tumorigenic descendants ( Fig. 2d ). Figure 2e shows that in Sox2-depleted cells not only is YAP protein expression decreased, but a much higher proportion of phosphorylated (transcriptionally inactive) YAP is detected, again indicating activation of the Hippo pathway in Sox2-depleted cells Accordingly, YAP is mostly nuclear in parental OS cells, while it is found mainly in the cytoplasm in Sox2-depleted cells ( Supplementary Fig. 3 ). Osteosarcoma stem cells have high YAP, low Nf2 and WWC1 As previously reported, the mOS cell lines used in this work contain a sizeable portion of cells capable of forming spheres in suspension culture in serum-free medium (osteospheres), thought to represent a population of tumour initiating CSC [12] . Such osteospheres are enriched in Sox2 expression and other stem cell markers, such as Sca-1. We determined the expression of YAP, WWC1 and Nf2 in the osteospheres and found that, similarly to Sox2, YAP was overexpressed, while Nf2 and WWC1 were downregulated when compared with the total adherent population ( Fig. 3a ). 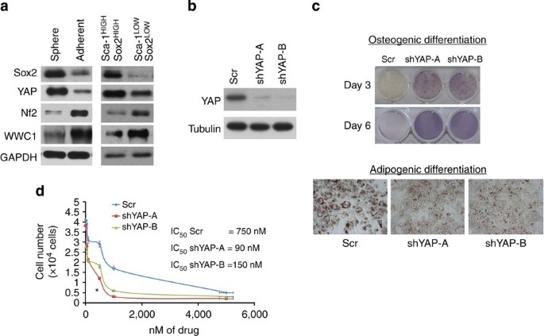Figure 3: YAP expression marks a population of osteosarcoma stem cells. (a) Western analysis of Sox2, YAP, Nf2 and WWC1 in osteosphere-forming cells and adherent cultures (left panel) and Sca-1High/Sox2Highversus Sca-1LowSox2Lowcells (right panel) from mOS-482 cells. (b) Western analysis of YAP in mOS-482 cells expressing scrambled or two independent YAP shRNAs (shRNA-A and shRNA-B). (c) Osteogenic and adipogenic differentiation assay. mOS-482 cells expressing scrambled or YAP shRNA-A/B were plated in either osteogenic or adipogenic medium. Osteogenic differentiation was detected using alkaline phosphatase staining. Adipogenesis was detected by Oil Red O staining of cells induced for 15 days (magnification × 100). Results from representative plates at the indicated times are shown. (d) mOS-482 cells expressing scrambled or YAP shRNAs were grown in increasing doses of methotrexate for 48 h and surviving cell populations were counted. IC50values are shown in the inset. Figure 3: YAP expression marks a population of osteosarcoma stem cells. ( a ) Western analysis of Sox2, YAP, Nf2 and WWC1 in osteosphere-forming cells and adherent cultures (left panel) and Sca-1 High /Sox2 High versus Sca-1 Low Sox2 Low cells (right panel) from mOS-482 cells. ( b ) Western analysis of YAP in mOS-482 cells expressing scrambled or two independent YAP shRNAs (shRNA-A and shRNA-B). ( c ) Osteogenic and adipogenic differentiation assay. mOS-482 cells expressing scrambled or YAP shRNA-A/B were plated in either osteogenic or adipogenic medium. Osteogenic differentiation was detected using alkaline phosphatase staining. Adipogenesis was detected by Oil Red O staining of cells induced for 15 days (magnification × 100). Results from representative plates at the indicated times are shown. ( d ) mOS-482 cells expressing scrambled or YAP shRNAs were grown in increasing doses of methotrexate for 48 h and surviving cell populations were counted. IC 50 values are shown in the inset. Full size image We then fractionated our mOS cells into Sca-1 High and Sca-1 Low fractions, by magnetic fractionation and FACS sorting. Sca-1 High cells are also Sox2 High , while Sca-1 Low cells express low levels of Sox2, as previously described [12] . The Sox2 High , Sca-1 High fraction contains the tumour-initiating portion of the total cell population ( Table 1 ). Sca-1 High , Sox2 High cells showed high YAP expression and low Nf2 and WWC1 expression, and the reverse was seen in Sca-1 Low Sox2 Low cells ( Fig. 3a ). The mRNA for these genes was similarly regulated in these cell populations ( Supplementary Fig. 4a,b ). Knockdown of YAP expression by shRNA in mOS-482 cells ( Fig. 3b ) greatly reduced their ability to form osteospheres in a limiting dilution assay ( Table 2 ), while YAP overexpression in primary osteoblasts increased sphere formation ( Supplementary Fig. 5 ). Expression of bona fide YAP target genes were also reduced in YAP-knockdown osteosarcoma cells ( Supplementary Fig. 4c ) Table 1 Limiting dilution analysis (LDA) for tumorigenicity of Sca-1 High and Sca-1 Low cells fractionated from mOS-482 cells. Full size table Table 2 Limiting dilution analysis for secondary sphere formation of mOS-482 cells expressing scrambled or shYAP lentivirus. Full size table A hallmark of CSCs from mesenchymal tumours is multipotency—the ability to differentiate into multiple lineages [9] . To determine whether YAP expression marks a multipotent CSC fraction, we tested the ability of YAP-depleted cells to undergo osteogenic or adipogenic differentiation. Knockdown of YAP increased osteogenic differentiation, and decreased adipogenic differentiation, a behaviour similar to that of Sox2-depleted cells ( Fig. 3c ). This conclusion was confirmed by determining the increased or decreased expression of genes characteristic of osteogenic or adipogenic differentiation, respectively ( Supplementary Fig. 6a ). In contrast, overexpression of YAP in primary osteoblasts inhibited osteogenesis ( Supplementary Fig. 5 ). Using a limiting dilution analysis, we showed that the tumorigenicity of the YAP knockdown cells was significantly reduced ( Table 3 ). Consistent with the notion that CSC are more refractory to chemotherapeutic agents, YAP depletion sensitized osteosarcoma cells to methotrexate, a first line of chemotherapy in osteosarcoma ( Fig. 3d ). Thus, these results identify high YAP, low Nf2 and low WWC1 expression as markers of osteosarcoma stem cells and confirm the notion that YAP is a direct Sox2 target and effector, as its expression parallels that of Sox2 and its overexpression or knockdown mimics the results obtained with Sox2 overexpression or depletion. Table 3 Limiting dilution analysis for tumorigenicity of mOS-482 cells expressing scrambled or shYAP lentivirus. Full size table Expression of Nf2 restores osteoblastic differentiation To determine whether Nf2 plays a role in YAP regulation in osteosarcoma, we expressed Nf2 in mOS-482 using a lentiviral system. Overexpression of Nf2 decreased YAP expression and osteosphere formation ( Fig. 4a ), while it increased osteogenesis and reduced adipogenesis ( Fig. 4a ; qPCR analysis— Supplementary Fig. 6b ). In contrast, knockdown of Nf2 by shRNA in primary osteoblasts increased YAP and inhibited osteogenic differentiation ( Fig. 4b ; qPCR analysis— Supplementary Fig. 6c ). The inhibition of YAP by Nf2 was dependent on the Hippo pathway kinases, Mst1/2 (ref. 36 ) and Lats1/2 as their depletion in Nf2-overexpressing cells resulted in increased YAP expression and sphere formation ( Fig. 4c ). The differentiation-inducing ability of Nf2 was overcome by overexpression of wild type (WT) and a YAP mutant resistant to phosphorylation YAP(5SA) [26] ( Fig. 4d ; qPCR analysis— Supplementary Fig. 6d ). Conversely, a YAP mutant deficient in TEAD binding YAP(94SA) [26] was unable to overcome the differentiation-inducing effect of Nf2. Interestingly, YAP(94SA) restores osteogenic differentiation in the control cells ( Fig. 4d ). Taken together, these data confirm that Nf2 restrains YAP activity primarily via the Hippo pathway. 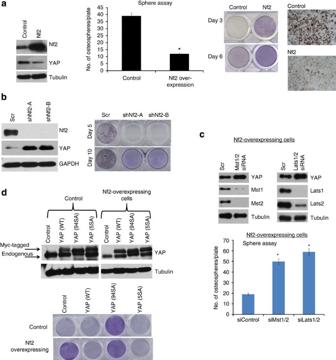Figure 4: Nf2 is required for osteogenic differentiation of osteosarcomas. (a) Nf2 overexpression in mOS-482 cells increases osteogenic differentiation. Western analysis of Nf2 expression mOS-482 cells transduced with a control or Nf2 retrovirus (left panel). Osteosphere assay (middle panel), and osteogenic and adipogenic differentiation (right panel). *P<0.05 byt-test. Error bars represent mean ± s.d. (b) Nf2 depletion in primary osteoblasts reduces osteogenic differentiation. Analysis of Nf2 in primary osteoblasts transduced with scrambled or two independent shNf2 lentivirus- shNf2-A and shNf2-B. Western analysis (left panel). Osteogenic differentiation (right panel). (c) Depletion of Mst1/2 or Lats1/2 in Nf2-overexpressing cells restores sphere formation. Nf2-overexpressing mOS-482 cells were transfected with control (scrambled) or Mst1/2 siRNAs or Lats1/2 siRNAs. Western analysis (upper panel) and sphere assay (lower panel). *P<0.05 byt-test. Error bars represent mean ± s.d. (d) Control or Nf2-overexpressing mOS-482 cells were transduced with myc-tagged YAP (WT), YAP (5SA—constitutively active YAP mutant) or YAP (94SA—YAP mutant deficient in TEAD-binding) retroviruses. Western analysis (upper panel). Osteogenic differentiation (lower panel). Figure 4: Nf2 is required for osteogenic differentiation of osteosarcomas. ( a ) Nf2 overexpression in mOS-482 cells increases osteogenic differentiation. Western analysis of Nf2 expression mOS-482 cells transduced with a control or Nf2 retrovirus (left panel). Osteosphere assay (middle panel), and osteogenic and adipogenic differentiation (right panel). * P <0.05 by t -test. Error bars represent mean ± s.d. ( b ) Nf2 depletion in primary osteoblasts reduces osteogenic differentiation. Analysis of Nf2 in primary osteoblasts transduced with scrambled or two independent shNf2 lentivirus- shNf2-A and shNf2-B. Western analysis (left panel). Osteogenic differentiation (right panel). ( c ) Depletion of Mst1/2 or Lats1/2 in Nf2-overexpressing cells restores sphere formation. Nf2-overexpressing mOS-482 cells were transfected with control (scrambled) or Mst1/2 siRNAs or Lats1/2 siRNAs. Western analysis (upper panel) and sphere assay (lower panel). * P <0.05 by t -test. Error bars represent mean ± s.d. ( d ) Control or Nf2-overexpressing mOS-482 cells were transduced with myc-tagged YAP (WT), YAP (5SA—constitutively active YAP mutant) or YAP (94SA—YAP mutant deficient in TEAD-binding) retroviruses. Western analysis (upper panel). Osteogenic differentiation (lower panel). Full size image The Hippo pathway is a Sox2 downstream effector To further determine whether the Hippo pathway acts as a Sox2 downstream effector in osteosarcoma stem cell maintenance, we performed rescue experiments by overexpressing YAP or knocking down Nf2 and WWC1 expression in Sox2-depleted cells by siRNAs. Either YAP overexpression or Nf2/WWC1 depletion significantly restored the capacity of Sox2-depleted cells to form osteospheres, although not to the same levels observed in the parental osteosarcoma cells ( Fig. 5 ). Downregulation of Nf2 or WWC1 expression in Sox2-depleted cells was accompanied by increased YAP protein expression, in line with the notion that the Hippo pathway is an important downstream effector of Sox2 in osteosarcoma stem cells ( Fig. 5 ). 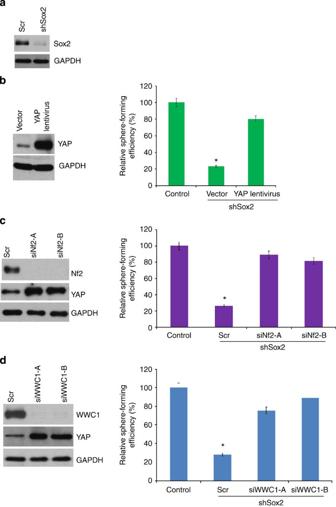Figure 5: YAP overexpression or Nf2/WWC1 depletion restores osteopheres in Sox2-depleted cells. (a) Western blot showing levels of Sox2 expression in mOS-482–shSox2 cells. (b) Western analysis of YAP expression in shSox2 cells transduced with a control or YAP lentivirus (left panel). Relative sphere-forming efficiency of YAP-transduced shSox2 cells compared with control (parental) mOS-482 cells (right panel). (c) Western analysis of YAP and Nf2 expression in shSox2 cells transfected with scrambled (scr) or two independent Nf2 siRNAs (left panel). Relative sphere-forming efficiency of Nf2-depleted shSox2 cells compared with control (parental) mOS-482 cells (right panel). (d) Western analysis of YAP and WWC1 expression in shSox2 cells transfected with scrambled (scr) or two independent WWc1 siRNAs (left panel). Relative sphere-forming efficiency of WWC1-depleted shSox2 cells compared with control (parental) mOS-482 cells (right panel). *P<0.05 by ANOVA. Error bars represent mean ± s.d. Figure 5: YAP overexpression or Nf2/WWC1 depletion restores osteopheres in Sox2-depleted cells. ( a ) Western blot showing levels of Sox2 expression in mOS-482–shSox2 cells. ( b ) Western analysis of YAP expression in shSox2 cells transduced with a control or YAP lentivirus (left panel). Relative sphere-forming efficiency of YAP-transduced shSox2 cells compared with control (parental) mOS-482 cells (right panel). ( c ) Western analysis of YAP and Nf2 expression in shSox2 cells transfected with scrambled (scr) or two independent Nf2 siRNAs (left panel). Relative sphere-forming efficiency of Nf2-depleted shSox2 cells compared with control (parental) mOS-482 cells (right panel). ( d ) Western analysis of YAP and WWC1 expression in shSox2 cells transfected with scrambled (scr) or two independent WWc1 siRNAs (left panel). Relative sphere-forming efficiency of WWC1-depleted shSox2 cells compared with control (parental) mOS-482 cells (right panel). * P <0.05 by ANOVA. Error bars represent mean ± s.d. Full size image Nf2 and WWC1 are directly repressed by Sox2 ChIP-PCR experiments in osteosarcoma cells show that Sox2 binds the same sites in the YAP 5′ region observed in osteoprogenitor cells, indicating that Sox2 targets the YAP gene also in this tumour (not shown). Accordingly, YAP mRNA was elevated in osteosphere-forming cells and in Sox2 High cells as compared with Sox2 Low cells ( Supplementary Fig. 4a,b ), but was not strongly decreased by Sox2 depletion ( Supplementary Fig. 7 ; see discussion). ChIP-Seq analysis also identified two prominent Sox2-binding regions, one upstream of the Nf2 transcription start site ( Fig. 6a ) and the other 3′ of WWC1 ( Fig. 7a ). Consistent with the microarray analysis, both genes are upregulated at the mRNA and protein level in mOS cells depleted of Sox2 by shRNA. Nf2 mRNA is increased 3-fold and WWC1 is increased 4.5-fold in Sox2-depleted cells ( Figs 6b and 7b ). 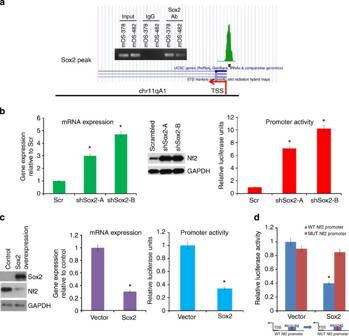Figure 6: Sox2 negatively regulates Nf2 by binding to its promoter region. (a) Sox2 binds to the Nf2 5′ region. Sox2 ChIP-Seq shows one peak (green) of Sox2-bound genomic sequence in the Nf2 5′ region in Sox2-overexpressing osteoprogenitors29. Inset shows validation of ChIP-Seq in osteosarcoma cells by PCR analysis using primers flanking the Sox2-binding site in the Nf2 5′ region. (b) Analysis of Nf2 expression in mOS-482 cells expressing scrambled or two independent Sox2 shRNAs-A and B. Left panel: Nf2 mRNA expression normalized to actin levels. Middle panel: western analysis of Nf2 expression. Right panel: luciferase assay. A 1.5-kb fragment of the Nf2 promoter containing the Sox2-binding site was cloned into a pGL3-Basic luciferase vector. Activity of the Nf2 5′UTR luciferase reporter construct was normalized to Renilla luciferase activity. *P<0.05 byt-test. Error bars represent mean ± s.d. (c) Analysis of Nf2 expression in primary osteoblasts cells expressing control or Sox2 lentivirus. Left panel—Western analysis of Nf2 expression. Middle panel—Nf2 mRNA expression normalized to actin levels. Right panel—Luciferase assay. Activity of the Nf2 5′UTR luciferase construct was normalized to Renila luciferase activity. *=P<0.05 byt-test. Error bars represent mean ± s.d. (d) Sox2 binding is required for suppression of Nf2 expression. The Nf2 5′ promoter region has one Sox2-binding site. This was mutated in the Nf2 luciferase construct (used inb) and luciferase activity was measured and normalized to Renilla activity. *P<0.05 byt-test. Error bars represent mean ± s.d. WT=wild-type promoter, MUT=promoter with a mutant Sox2-binding site. The mutated sites are shown in red in the schematic. Figure 6: Sox2 negatively regulates Nf2 by binding to its promoter region. ( a ) Sox2 binds to the Nf2 5′ region. Sox2 ChIP-Seq shows one peak (green) of Sox2-bound genomic sequence in the Nf2 5′ region in Sox2-overexpressing osteoprogenitors [29] . Inset shows validation of ChIP-Seq in osteosarcoma cells by PCR analysis using primers flanking the Sox2-binding site in the Nf2 5′ region. ( b ) Analysis of Nf2 expression in mOS-482 cells expressing scrambled or two independent Sox2 shRNAs-A and B. Left panel: Nf2 mRNA expression normalized to actin levels. Middle panel: western analysis of Nf2 expression. Right panel: luciferase assay. A 1.5-kb fragment of the Nf2 promoter containing the Sox2-binding site was cloned into a pGL3-Basic luciferase vector. Activity of the Nf2 5′UTR luciferase reporter construct was normalized to Renilla luciferase activity. * P <0.05 by t -test. Error bars represent mean ± s.d. ( c ) Analysis of Nf2 expression in primary osteoblasts cells expressing control or Sox2 lentivirus. Left panel—Western analysis of Nf2 expression. Middle panel—Nf2 mRNA expression normalized to actin levels. Right panel—Luciferase assay. Activity of the Nf2 5′UTR luciferase construct was normalized to Renila luciferase activity. *= P <0.05 by t -test. Error bars represent mean ± s.d. ( d ) Sox2 binding is required for suppression of Nf2 expression. The Nf2 5′ promoter region has one Sox2-binding site. This was mutated in the Nf2 luciferase construct (used in b ) and luciferase activity was measured and normalized to Renilla activity. * P <0.05 by t -test. Error bars represent mean ± s.d. WT=wild-type promoter, MUT=promoter with a mutant Sox2-binding site. The mutated sites are shown in red in the schematic. 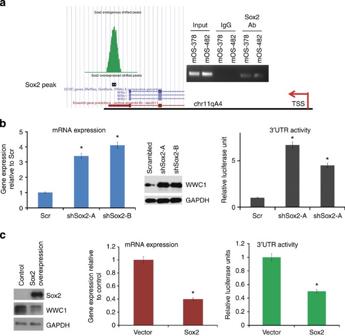Figure 7: Sox2 negatively regulates WWC1 by binding to its 3′UTR. (a) Sox2 binds to the WWC1 3′UTR. Sox2 ChIP-Seq shows one peak (green) of Sox2-bound genomic sequence in the WWC1 3′UTR in SOX2-overexpressing osteoprogenitors29. Inset shows validation of ChIP-Seq in osteosarcoma cells by PCR analysis using primers flanking the Sox2-bidning site in the WWC1 3′UTR. (b) Analysis of WWC1 expression in mOS-482 cells expressing scrambled or two independent Sox2 shRNAs- A and B. Left panel: WWC1 mRNA expression normalized to actin levels. Middle panel: western analysis of WWC1. Right panel: luciferase assay. A 800-bp fragment of the WWC1 3′UTR containing Sox2-binding sites was cloned downstream of the luciferase-coding region in the pTK vector. Activity of the WWC1 3′UTR luciferase construct was normalized to Renilla luciferase activity. *P<0.05 byt-test. Error bars represent mean ± s.d. (c) Analysis of WWC1 expression in primary osteopblasts cells expressing control or Sox2 lentivirus. Left panel: western analysis of WWC1. Middle panel: WWC1 mRNA expression normalized to actin levels. Right panel: luciferase assay. Activity of the WWC1 3′UTR luciferase construct was normalized to Renila luciferase activity. *P<0.05 byt-test. Error bars represent mean ± s.d. Full size image Figure 7: Sox2 negatively regulates WWC1 by binding to its 3′UTR. ( a ) Sox2 binds to the WWC1 3′UTR. Sox2 ChIP-Seq shows one peak (green) of Sox2-bound genomic sequence in the WWC1 3′UTR in SOX2-overexpressing osteoprogenitors [29] . Inset shows validation of ChIP-Seq in osteosarcoma cells by PCR analysis using primers flanking the Sox2-bidning site in the WWC1 3′UTR. ( b ) Analysis of WWC1 expression in mOS-482 cells expressing scrambled or two independent Sox2 shRNAs- A and B. Left panel: WWC1 mRNA expression normalized to actin levels. Middle panel: western analysis of WWC1. Right panel: luciferase assay. A 800-bp fragment of the WWC1 3′UTR containing Sox2-binding sites was cloned downstream of the luciferase-coding region in the pTK vector. Activity of the WWC1 3′UTR luciferase construct was normalized to Renilla luciferase activity. * P <0.05 by t -test. Error bars represent mean ± s.d. ( c ) Analysis of WWC1 expression in primary osteopblasts cells expressing control or Sox2 lentivirus. Left panel: western analysis of WWC1. Middle panel: WWC1 mRNA expression normalized to actin levels. Right panel: luciferase assay. Activity of the WWC1 3′UTR luciferase construct was normalized to Renila luciferase activity. * P <0.05 by t -test. Error bars represent mean ± s.d. Full size image The downregulation of Nf2 and WWC1 by Sox2 was intriguing, as Sox2 has generally been reported to act as a transcriptional activator. We therefore cloned the Nf2 promoter upstream of the luciferase reporter in the pGL3 basic vector and studied reporter expression in the presence or absence of Sox2. The luciferase activity of the Nf2 promoter region was higher in mOS cells expressing Sox2 shRNA ( Fig. 6b ). Conversely, overexpression of Sox2 by lentiviral transduction in primary osteoblasts results in substantial inhibition (approximately fourfold) of both the promoter reporter construct and endogenous Nf2 expression ( Fig. 6c ). Mutation of the single Sox2-binding site in the Nf2 promoter abolished the inhibitory effect of Sox2 ( Fig. 6d ). Thus, we conclude that Nf2 expression is directly transcriptionally repressed by Sox2. We have extended this analysis to WWC1 (Kibra), the second Hippo pathway activator that appears to be repressed by Sox2. Sox2 binds to the WWC1 3′ region, within the 3′ untranslated portion of WWC1 mRNA ( Fig. 7a ). Because of this unusual location we thought it necessary to demonstrate that the Sox2-binding element in the 3′ region of the WWC1 gene behaves as a silencing element, which is repressed by Sox2. We therefore cloned the putative WWC1 silencer downstream of the luciferase gene in the pTK plasmid, and tested the activity of this plasmid in cells expressing high or low levels of Sox2. Similarly to the results obtained with Nf2, Sox2 knockdown increased, and high Sox2 expression inhibited the activity of the WWC1 3′UTR reporter. Thus, we conclude that WWC1 expression is also downregulated by Sox2 through its interaction with a 3′ regulatory element ( Fig. 7 ). The Sox2-Hippo axis is conserved in multiple cell types Our studies thus far establish that Sox2 represses the Hippo pathway in osteosarcoma cells in part through transcriptional inhibition of two activators—Nf2 and WWC1. To test whether this holds true in other cellular contexts, we used NIH-3T3 cells, an immortalized murine fibroblastic cell line that does not express endogenous Sox2. We established a stable NIH-3T3 line that expresses Sox2. As seen in Fig. 8a , overexpression of Sox2 suppresses Nf2 and WWC1 expression with a concurrent increase in YAP expression (qPCR mRNA analysis in Supplementary Fig. 8 ). Sox2-overexpressing NIH-3T3 cells also proliferate significantly faster than the control cells ( Fig. 8a ). Depletion of Nf2 in NIH-3T3 cells using shRNA mimics Sox2 overexpression both in increased YAP expression and proliferative ability. To confirm whether this Hippo-suppressive role of Sox2 operates in another cancer cell type that has high levels of endogenous Sox2 and requires Sox2 to maintain stemness, we knocked down Sox2 in primary human cultures of GBM that express high levels of Sox2 and differentiate on Sox2 depletion. In these cells, sphere formation was markedly decreased by Sox2 knockdown [37] . We also found that depletion of Sox2 decreases YAP and increases Nf2 expression, consistent with the notion that Sox2 antagonizes the Hippo pathway ( Fig. 8b ). In addition, when we differentiated these cultures with serum, we saw a decrease in Sox2 expression with a concurrent induction of Nf2 and GFAP, which marks differentiated astrocytes ( Fig. 8c ). Thus, these studies in NIH-3T3 and GBM cells demonstrate that the Hippo-suppressive role of Sox2 resulting in unrestrained YAP activity is conserved in multiple cell types ( Fig. 8d ). 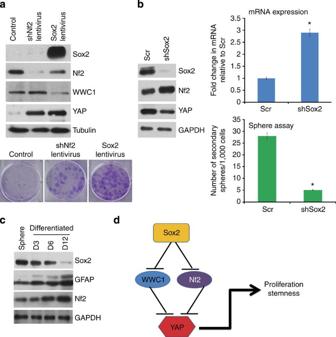Figure 8: The Sox2-Hippo axis is conserved in multiple cell types. (a) Upper panel: western analysis of YAP, WWC1, Nf2 and Sox2 in NIH-3T3 cells (control, or Nf2 shRNA-A lentivirus or Sox2 lentivirus). Lower panel: colony assay of NIH-3T3 cells expressing the indicated constructs. Colonies were stained with Crystal violet and counted after 10 days. (b) Primary glioblastoma multiforme (GBM) cells were transduced with a control or Sox2 shRNA lentivirus. Left panel: western analysis of Sox2, Nf2 and YAP. Upper right panel—Nf2 mRNA expression normalized to actin. Lower right panel- sphere assay. *P<0.05 byt-test. Error bars represent mean ± s.d. (c) Western analysis of Sox2, GFAP and Nf2 in primary GBM cells grown in sphere cultures (sphere) or differentiated for 3, 6 or 12 days (D3, D6 and D12, respectively). (d) Schematic of Sox2 regulation of Hippo pathway components. Sox2 represses Nf2 and WWC1 that restrain YAP transcriptional function. Figure 8: The Sox2-Hippo axis is conserved in multiple cell types. ( a ) Upper panel: western analysis of YAP, WWC1, Nf2 and Sox2 in NIH-3T3 cells (control, or Nf2 shRNA-A lentivirus or Sox2 lentivirus). Lower panel: colony assay of NIH-3T3 cells expressing the indicated constructs. Colonies were stained with Crystal violet and counted after 10 days. ( b ) Primary glioblastoma multiforme (GBM) cells were transduced with a control or Sox2 shRNA lentivirus. Left panel: western analysis of Sox2, Nf2 and YAP. Upper right panel—Nf2 mRNA expression normalized to actin. Lower right panel- sphere assay. * P <0.05 by t -test. Error bars represent mean ± s.d. ( c ) Western analysis of Sox2, GFAP and Nf2 in primary GBM cells grown in sphere cultures (sphere) or differentiated for 3, 6 or 12 days (D3, D6 and D12, respectively). ( d ) Schematic of Sox2 regulation of Hippo pathway components. Sox2 represses Nf2 and WWC1 that restrain YAP transcriptional function. Full size image Mounting evidence suggests that Sox2 marks and maintains CSC in a variety of cancers [38] , including tumours of epithelial (for example, the lung, skin, oesophageal and gastric) [39] , [40] , neural [41] and mesenchymal (for example, Ewing’s sarcoma) [42] origin. This is not simply a reflection of the stem-like nature of these cells as other stem cell transcription factors (for example, Oct4) are not expressed in CSC from osteosarcomas [43] . It is therefore of great interest to understand not only how the expression of this stem cell transcription factor is maintained or activated in CSC, but also the mechanisms by which Sox2 expression induces or maintains a CSC phenotype. In this report we highlight a previously unidentified mechanism through which Sox2 maintains a stem cell phenotype in the mesenchymal tumour osteosarcoma. We show here that Sox2 antagonizes the tumour-suppressive Hippo pathway by directly regulating key genes in the pathway. Furthermore, the Sox2-dependent repression of the Hippo pathway is conserved in other cellular contexts. These findings identify a novel key mechanism through which this transcription factor determines the phenotype of CSC. As the Hippo pathway is tumour suppressive in a variety of cancers [31] , [44] , [45] , [46] , [47] , we analysed the activity of this pathway in osteosarcomas, mesenchymal tumours in which we had previously shown a dependence on Sox2 for the maintenance of tumour-initiating CSC. YAP, a downstream Hippo effector, is directly regulated by Sox2 in MSC and osteoprogenitors [29] . Its overexpression inhibited osteogenic differentiation and could preserve ‘stemness’ and viability in Sox2-null MSC or osteoprogenitors, identifying it as a key Sox2 target gene. Overexpression of YAP can antagonize the repressive Hippo pathway by overcoming the activity of the Lats kinases, which phosphorylate and inactivate YAP. By examining the gene expression profiles of two mouse lines of osteosarcomas and that of their Sox2-depleted, no longer tumorigenic, derivatives, we found that two Hippo pathway activators, Nf2 (Merlin) and WWC1 (Kibra), were expressed at very low levels in the parental cells and strongly upregulated in the Sox2-depleted derivatives. This finding was recapitulated in human osteosarcoma cells as well ( Supplementary Fig. 9 ). YAP protein was highly expressed in the parental cells and downregulated in Sox2-depleted cells. Meta analysis of a large panel of human osteosarcomas confirmed the widespread upregulation of YAP and the downregulation of Nf2 and WWC1 in such tumours. These results suggested that the Hippo pathway, which represses the transcriptional activity of the YAP cofactor, was antagonized in osteosarcomas in a Sox2-dependent manner. Accordingly, the expression of a YAP/TEAD-responsive reporter plasmid, as well as that of YAP/TEAD target genes, was high in the parental mOS cell and low in Sox2-depleted cells, while the proportion of phosphorylated (inactive) YAP was much higher in the Sox2-depleted cells. TAZ, the YAP paralogue, was also elevated in osteosarcoma cells, but not as consistently as that of YAP. TAZ does not appear to be a direct Sox2 target, and its expression is not decreased in Sox2-depleted cells [29] . Furthermore, TAZ stimulates osteogenic differentiation through Runx2 activation, whereas YAP suppresses Runx2-mediated gene transcription [48] , [49] , [50] . In fact, most of the cell lines used in this work have negligible levels of TAZ expression ( Supplementary Fig. 2a ). In osteosarcoma cells coexpressing TAZ and YAP, TAZ is unable to maintain osteospheres following YAP depletion ( Supplementary Fig. 2b ). Thus, although TAZ plays a role in breast CSC [51] , it appears not to compensate for YAP depletion in osteosarcoma. We therefore focused our studies on YAP. To test the hypothesis that inhibition of the Hippo pathway was a key property of osteosarcoma stem cells, we examined YAP, WWC1 and Nf2 expression in the CSC, tumour-initiating fraction of osteosarcomas. We also examined the effect of Hippo pathway activation or downregulation on the ability of osteosarcoma cells to form tumours, osteospheres, and differentiate into the osteoblastic or adipocytic lineage. The Sox2 High , Sca-1 High tumour-initiating fraction of the OS cell population or the osteosphere-forming cells showed high YAP and reduced Nf2 and WWC1 expression, and this pattern was reversed in the Sca-1 Low , Sox2 Low fraction or in adherent cells. ShRNA depletion of YAP or overexpression of Nf2 in two mOS cell lines depletes the tumour-initiating population, as evidenced by decreased sphere-forming ability and increased commitment to the osteogenic fate. Importantly, the differentiation-inducing effects of Nf2 observed were dependent on the Hippo pathway kinases, as depletion of Mst1/2 or Lats1/2 abolished the effects of Nf2 on YAP expression and function. While Nf2 has Hippo-independent and dependent roles [19] , its tumour-suppressive role and effect on YAP seem to occur primarily through activation of the Hippo kinase cascade. In summary, we conclude that downregulation of the Hippo pathway is a hallmark of osteosarcoma CSC, and that subverting this downregulation inhibits tumour initiation and allows osteogenic differentiation, mimicking the effects of Sox2 depletion, and thus identifying YAP, Nf2 and WWC1 as key targets of Sox2. These results suggest that activation of the Hippo pathway could be a novel type of intervention for the treatment of these tumours. In fact, YAP depletion by shRNA or disruption of the YAP-TEAD transcriptional complex by verteporfin sensitizes to cells to methotrexate, suggesting that inhibition of YAP-dependent gene expression can deplete the CSC fraction of osteosarcomas (data not shown). YAP overexpression has been associated with a variety of cancers and metastatic disease in both humans and mice [52] , [53] , [54] , [55] . While Sox2 binds to the YAP promoter both in osteoprogenitors and osteosarcoma cells, and can strongly increase the activity of a YAP reporter plasmid, the expression of YAP mRNA was not significantly reduced in Sox2-depleted osteosarcoma cells. The two mOS cell lines used in this study show amplification of a large segment of chromosome 9 that includes the YAP gene (data not shown). Amplifications of syntenic regions have been reported for chromosome 11 in human osteosarcoma [46] , [56] . We therefore consider very likely that the effect of Sox2 on YAP transcription, which is marked in osteoprogenitors, was not striking in osteosarcomas as amplification of the YAP gene would reduce the extent of Sox2 transcriptional dependency. In contrast, the expression of YAP protein is strongly reduced both in Sox2-depleted osteosarcoma cells, and in the non-CSC fraction. We believe that this is the result of the upregulation of the two Hippo activators, Nf2 and WWC1, that leads to increased phosphorylation of YAP, cytoplasmic retention and proteolytic degradation. Thus, in osteosarcomas, YAP expression is stimulated by Sox2 possibly through a minor transcriptional effect that is amplified by increased YAP protein stability. Chan et al. [57] have recently shown that YAP induction via Hedgehog signalling is important for the tumorigenic properties of osteoblastic osteosarcoma. As Hedgehog is reported to be a downstream mediator of Sox2 function in neural stem cells [58] , this may represent an additional mechanism by which Sox2 maintains YAP expression. Of the two Hippo activators that we found deregulated in osteosarcomas, less is known about WWC1’s potential involvement in cancer. A recent report suggests that WWC1 activation of the Hippo pathway in breast cancer cells can suppress EMT [59] , and the Drosophila homologue, KIBRA, functions as a tumour suppressor [31] . In contrast, Nf2 mutations are responsible for neurofibromatosis type 2, which is characterized by multiple neuromas, meningiomas and schwannomas [60] . Furthermore, multiple somatic mutations have been reported for Nf2 , mostly in meningiomas, and peripheral nerve tumours, and Nf2 heterozygous mice develop a high frequency of metastatic tumours, particularly osteosarcomas and liver carcinomas, identifying Nf2 as a bone fide tumour suppressor gene [61] . In addition to its role in activating upstream components of the Hippo pathway, Nf2 can also accumulate in the cell nucleus to inhibit the activity of the DCAF1 E3 ubiquitin ligase, a function that appears to be important for its tumour-suppressing activity [62] . DCAF1 ubiquitinates and therefore inhibits the Lats1/2 kinases. Low Nf2 expression would increase E3 ubiquitin ligase activity and target Lats1/2 for degradation, thus promoting YAP-driven transcription and tumorigenesis [63] . In this model, Nf2 would activate the Hippo pathway at least at two distinct levels, by promoting the formation of upstream complexes and by increasing the stability of the Lats1/2 kinases. It has also been reported that expression of Nf2 in Rb-deficient mOS restores osteoblastic differentiation through an interaction with ERM proteins that restores cell adhesion [64] . In conclusion, the simultaneous regulation of two genes in the Hippo pathway provides a convergent effect on pathway inactivation in osteosarcomas. A striking feature of our findings is that both positive regulators of the Hippo pathway, (Nf2 and WWC1) and the downstream effector YAP, appear to be directly regulated by Sox2. They all show distinct Sox2 peaks by Chip-Seq experiments, corresponding to CpG islands and/or DNase hypersensitivity sites. All three genes are affected by Sox2 abundance. We previously reported the direct induction of YAP transcription by Sox2 in MSCs and osteoprogenitors [29] . The putative Sox2 repressive regulatory elements of WWC1 and Nf2 were more intriguing, as Sox2 has been generally considered a transcriptional activator. We thus cloned DNA segments around the Sox2-binding sites for both genes in reporter plasmids and showed they could be directly repressed by Sox2 in coexpression experiments and that mutations in the Sox2-binding sites abolished repression. We also conclusively showed that the levels of endogenous WWC1 and Nf2 mRNAs were downregulated by Sox2 overexpression and upregulated by Sox2 depletion. Our findings are especially interesting in light of the fact that non-mutational mechanisms of Nf2 downregulation in tumours have not been previously described. It is well established that transcription factors can act as activators or repressors, depending on the cofactor with which they interact, interaction that can be determined by the flanking DNA sequence, cofactor abundance and also by the sequence of the transcription factor binding site, which leads to a different conformation of the bound transcription factor. It is interesting to note that Sox2 is generally thought to act in synergy with other transcription factors, which bind near the Sox2-binding site, the best known case being the Sox2/Oct4 interaction, which governs the expression of many ES cell genes [65] . Although expression of Oct4 in osteosarcoma cells has been reported, this finding does not appear reproducible [43] . We have never been able to detect Oct4 expression in the osteoblast lineage or in osteosarcomas, thus the manner by which Sox2 activates or represses gene transcription in these cells may require an interaction with multiple cofactors. A recent report has demonstrated that Sox2 can interact with the NuRD-HDAC-containing repressor complex and repress genes in ES cells to regulate pluripotency [66] . Thus, while traditionally considered a transcriptional activator, Sox2 can activate or inhibit gene expression in a context-dependent manner. Finally, we show that the ability of Sox2 to regulate YAP and Nf2 is maintained in other tumours, such as glioblastoma, and in cells which normally do not express Sox2, such as NIH-3T3 fibroblasts, suggesting a conserved mechanism of regulation among different cell lineages and pathologies. This Sox2-Hippo axis that maintains CSCs could serve as a target for cancer therapy. Cell culture The human osteosarcoma cell line U-2OS was obtained from the American Type Culture Collection. The OS-187 cells were a gift from Dr Nancy Gordon, from M.D. Anderson Cancer Center, Texas. The OS-99-1 cells were obtained from Dr Sheila Nielsen-Priess from University of Montana, Missoula. The parental Saos-2 cells and the Saos-2-LM7 cells (metastatic variant) were provided by Dr Eugenie Kleinerman, Anderson Cancer Center, Houston [67] . The mOS cell lines used in this study (mOS-482, mOS-379, mOS-648 and mOS-202M) and their derivatives (expressing scrambled or Sox2 shRNA) have been previously described [15] . All cells were maintained in DMEM supplemented with 10% fetal bovine serum. Cell lines expressing Nf2, Nf2 and YAP shRNA, and mutant YAP, were developed by infecting mOS cells with the specific virus and selecting with 4 μg ml −1 Puromycin, 500 μg ml −1 Hygromycin or both. Primary GBM cultures Following consent, fresh surgical specimens, classified as GBM based on WHO criteria, were collected from patients undergoing surgery in NYU Langone Medical Center in accordance with NYU’s Institutional Review Board (IRB) regulations (IRB# S12-01130). Within 1–2 h after surgical resection, tumours were enzymatically dissociated into single cells (Accutase, Innovative Cell Technologies). GBM cells were cultured in suspension in NSC media consisting of Neurobasal media (Life Technologies), N2 and B27 (without vitamin A) supplements ( × 1, Life Technologies), 20 ng ml −1 of human recombinant EGF (Life Technologies) and bFGF (R&D Systems). For differentiation assays, primary tumorsphere cultures were dissociated and plated as adherent cultures, which were maintained in Dulbecco’s Minimal Essential Media (DMEM, Life Technologies) and 10% fetal bovine serum (FBS, Life Technologies). Expression vectors, cloning and lentivirus production A 1.5-kb promoter region of the murine Nf2 promoter containing the Sox2-binding site was cloned into the HindIII site of the pGL3-Basic Vector (Promega, WI, USA). The Sox2-binding site in the Nf2 promoter was mutated using the Quick Change II Site-Directed Mutagenesis Kit from Agilent technologies, Santa Clara, CA. A 750-bp fragment of the 3′UTR of the murine WWC1 gene was cloned into the XbaI site of the pTK-Luciferase plasmid. The 8X-GTIIC TEAD luciferase reporter was a kind gift from Dr Stefano Piccolo. Nf2 shRNAs (mouse), Sox2 shRNAs (human) and YAP shRNAs (mouse) lentivirus were purchased from Sigma, St Louis, MO. The Nf2 lentivirus was a kind gift from Dr Filippo Giancotti. The FUCRW-Sox2 and FUCRW-YAP lentiviruses have been previously described [29] . Other retrovirus such as Myc-tagged WT YAP (Addgene # 33091), 5SA YAP (Addgene # 33093)and 94SA YAP (Addgene # 33094) all in the pQCXIH vector from the laboratory of Dr Kung-Lian Guan, and pBabe-Nf2 (Addgene # 14116) from the laboratory of Dr Tyler Jacks, were obtained from Addgene, Cambridge, MA. All lentiviruses used in this study were produced in 293T cells using pVSV-G, pLP1 and pLP2 as helper plasmids. All retroviruses were produced in 293-GP cells and pseudotyped with VSV-G. Microarray experiment Total cellular RNA from mOS482 and mOS-378 cells expressing either scrambled or Sox2 shRNA was extracted as previously described [68] . In brief, total cellular RNA was extracted by RNEASY Kit (Qiagen, Valencia, CA). RNA quality was assessed using an Agilent 2100 Bioanalyzer and Nanodrop ND-1000. cRNA was prepared from 100 ng RNA using the Affymetrix 3′ IVT Express labelling kit and array processing protocol (Affymetrix). cRNAs were hybridized to mouse genome 430A 2.0 arrays (Affymetrix), which contain 22,690 gene probes. Arrays were processed and scanned at New York University School of Medicine, Genome Technology Center according to procedures recommended by the manufacturer (Affymetrix). The microarray data have been deposited in GEO Database under Accession Number GSE64965 Sox2 ChIP-Seq in osteoprogenitors and gene expression analysis OB1 osteoprogenitor cells were transduced with either a control or Sox2-lentivirus and chromatin was prepared. ChIP-Seq analysis of Sox2 target genes has been previously described [29] . Antibodies are described in Supplementary Information . Quantitative RT-PCR using specific primers was performed as described [69] . Sequences of primers are available in Supplementary Information . Luciferase activity of all reporters was measured by the Stop and Glo Luciferase Assay Kit (Promega, WI). Limiting dilution analysis for CSC Decreasing concentrations of mOS-482 cells expressing either scrambled of shYAP were plated in defined N2B27 medium. Wells forming spheres after 12–14 days were scored as positive and data were analysed using the ELDA software. For limiting dilution analysis of tumorigenicity, decreasing concentrations of mOS-482 cells expressing either scrambled of shYAP were injected subcutaneously into 6- to 8-week-old female NOD/SCID mice. Tumour growth was monitored bi-weekly. All tumorigenesis studies were performed at the Antitumor Assessment Facility at Memorial Sloan Kettering Cancer Center under IACUC Approved Protocol Number A3311-01. Osteogenic and adipogenic differentiation Osteosarcoma cell lines were plated at a density of 50,000 cells per well of 24-well plates or 0.5 × 10 6 cells per well of six-well plates, and osteogenic or adipogenic differentiation was carried out as previously described [12] . Mice colony The spontaneous mouse model for osteosarcoma has been previously described [15] and obtained from Dr Stuart Orkin. Tumours were isolated from 3-month-old p53 Flox/Flox /Rb Flox/Flox /Osterix-Cre mice. All experiments were conducted at the New York School of Medicine Animal Facility under the approved IUCAC Protocol 140114-02. Western blotting For protein expression analysis, cells were grown to 80% confluence and lysed in RIPA buffer supplemented with protease and phosphatase inhibitors. Lysates were resolved on sodium dodecyl sulfate–PAGE (SDS–PAGE) gels and probes using appropriate antibodies, described in Supplementary Information . Each experiment was repeated at least twice and representative cropped immunoblots are shown. Uncropped images of western blots are included in Supplementary Fig. 10 . Immunohistochemistry Paraffin-embedded sections of PFA-fixed tumours were stained with anti-Sox2 and anti-YAP polyclonal antibodies. HRP-conjugated anti-rabbit secondary antibodies were obtained from Vector Laboratories (Burlingame, CA) and detected according to the manufacturer’s protocol. How to cite this article: Basu-Roy, U. et al. Sox2 antagonizes the Hippo pathway to maintain stemness in cancer cells. Nat. Commun. 6:6411 doi: 10.1038/ncomms7411 (2015).